Metagenome-wide analysis of antibiotic resistance genes in a large cohort of human gut microbiota The human gut microbiota is a reservoir of antibiotic resistance genes, but little is known about their diversity and richness within the gut. Here we analyse the antibiotic resistance genes of gut microbiota from 162 individuals. We identify a total of 1,093 antibiotic resistance genes and find that Chinese individuals harbour the highest number and abundance of antibiotic resistance genes, followed by Danish and Spanish individuals. Single-nucleotide polymorphism-based analysis indicates that antibiotic resistance genes from the two European populations are more closely related while the Chinese ones are clustered separately. We also confirm high abundance of tetracycline resistance genes with this large cohort study. Our study provides a broad view of antibiotic resistance genes in the human gut microbiota. Antibiotic resistance in pathogenic bacteria has been presenting an increasing threat to human health during the last decade, and it is widely accepted that the antibiotic resistance development and spread in microbes can be largely attributed to the abuse and misuse of antibiotics. A direct correlation between antimicrobial use and the extent of antimicrobial resistance has been reported [1] . The human gut is inhabited by a large bacterial population, and this microbiota has a profound influence on human physiology and nutrition. Critical functions, including protection against epithelial cell injury [2] , regulation of host fat storage [3] and stimulation of intestinal angiogenesis [4] , are crucial for human health. However, there has been increasing attention paid to the gut microbiota as a reservoir for antibiotic resistance genes [5] . According to this concept, antibiotic resistance genes in the human gut bacteria cannot only be exchanged inside the gut microbiota but can also be transferred to other bacteria, even if the bacteria are just passing through the intestine. This situation represents a high risk with regard to the increased emergence of antibiotic-resistant human pathogenic bacteria [6] . Moreover, it has been shown that resistant bacteria can persist for years in the human gut, even under short-term antibiotic administration [7] . The antibiotic resistance genes in the human gut microbiota have been characterized via different methods, including the isolation of resistance strains, PCR using specific primers and macroarray analysis [8] , [9] . Recently, metagenomic expression libraries were used to functionally characterize antibiotic resistance genes from faecal samples, and a total of 210 genes in the gut microbiome were identified [10] . The researchers suggested that the extremely high diversity of antibiotic resistance genes in the human microbiome could contribute to the future emergence of antibiotic resistance in human pathogens. These studies have enriched our understanding of the human gut microbiota as a reservoir for antibiotic resistance genes. A large number of genes have already been reported to confer antibiotic resistance. Taking tetracycline as an example, a total of 46 tetracycline resistance (TcR) determinants have been identified, consisting of 30 efflux genes, 12 genes encoding ribosomal protection proteins, 3 enzymatic inactivators and 1 conferring resistance via an unknown mechanism ( http://faculty.washington.edu/marilynr/tetweb1.pdf ). A good summary of antibiotic resistance genes is presented in the Antibiotic Resistance Genes Database (ARDB), including a total of 23,137 antibiotic resistance genes, 380 resistance genotypes and 249 corresponding antibiotics (version 1.1) [11] , and this database has been widely used for gene annotation [12] , [13] , [14] , [15] , [16] . The BGI previously published a large-scale DNA sequencing data set from 124 intestinal samples from European adults and established a human microbiome gene catalogue of 3.3 million non-redundant bacterial genes [17] . We expand this non-redundant human gut microbiome gene set, also referred to as ‘prevalent genes’, to 4.1 million genes with the addition of recent sequencing data from 38 Chinese individuals. To obtain a broad overview of the antibiotic resistance genes in the human gut microbiota, we searched this gene set using BLAST (Basic Local Alignment Search Tool) search against the ARDB, and the antibiotic resistance gene profiles of individuals from three different countries, China, Denmark and Spain, were analysed comparatively. Our results indicate that the human gut harbours more antibiotic resistance genes than other environments. The antibiotic resistance genes in the three countries differ from each other on both abundance and single-nucleotide polymorphisms (SNPs). Chinese individuals harbour the highest abundance of antibiotic resistance genes while Danish show the lowest. TcR genes are the most abundant group of antibiotic resistance genes in all three countries. Human gut harbours more antibiotic resistance genes We established a set of 4.1 million human gut microbiome genes from sequencing data of 162 people, consisting of 85 Danish, 39 Spanish and 38 Chinese individuals, as previously described [17] . Next, we searched this gene set as well as eight environmental metagenome data sets for antibiotic resistance genes via BLAST search against the core set of 7,825 antibiotic resistance proteins from the ARDB. To determine a threshold for antibiotic resistance gene BLAST search, the UniProtKB/SwissProt database was used as test data. The receiver operating characteristic and precision/recall rate at different similarity cutoff levels were plotted ( Supplementary Fig. S1 ). As the precision remained to 99.1% at 80% similarity cutoff, and it decreased when lower similarity cutoff was applied, we select 80% similarity cutoff as preferred BLAST search criteria to ensure that the picked antibiotic resistance genes are true positives, while enduring the loss of antibiotic resistance genes with less similarity (Methods). By using such criteria, we found a total of 1,093 unique antibiotic resistance genes among 4.1 million gut genes. These antibiotic resistance genes account for 0.266‰ of the total human gut microbiome gene set. Compared with other natural environments, including soil, marine, lake, and so on, antibiotic resistance genes are clearly very much enriched in human gut microbiota ( Supplementary Table S1 ). Phylogenetic origins of antibiotic resistance genes To compare the microbial origin of antibiotic resistance genes with other gut genes, we assigned the 1,093 antibiotic resistance genes and the set of 4.1 million genes, respectively, to different taxa according to the NCBI taxonomy guidelines with the assistance of the MEGAN program. Between the antibiotic resistance genes and the gut gene set, different assignments at the phylum level were observed, that is, 52% versus 56%, 15% versus 31% and 32% versus 6% to Firmicutes , Bacteroidetes and Proteobacteria , respectively ( Supplementary Fig. S2 ). This inconsistency may suggest that antibiotic resistance genes are less prone to occur in Bacteroidetes but more prone to exist in Proteobacteria when compared with other genes. The resistance gene types in different countries are diverse We grouped the 1,093 gut antibiotic resistance genes into 149 different resistance gene types according to the ARDB, among which 95 were single-drug resistance gene types and 54 were multi-drug resistance types. Next, we mapped all of the antibiotic resistance genes to each individual in the different populations. Both the Chinese and Danish population harboured 133 resistance gene types, and the Spanish population harboured 128 gene types. Among the 162 human samples, one Chinese sample, NLM023, exhibited the highest number of resistance gene types (89), while a Danish sample, MH0049, possessed the lowest number of gene types (33). To avoid bias introduced by the absolute number, we further computed the gene type number of per gigabase pairs (Gb) sequence in each individual ( Supplementary Table S2 ). The results showed that the Chinese individuals harboured higher number of resistance gene types (29±6 per Gb) than that of Danish (13±6) and Spanish individuals (11±2) (Mann–Whitney test, P =4.0E−15 and 7.0E−14, respectively), suggesting that more diverse antibiotic resistance gene types are present in the Chinese population. Of the 149 resistance gene types, 19, 9 and 14 types were found in each sample in the Chinese, Danish and Spanish populations, respectively, and 9 types, Ant6ia, BacA, VanRA, VanRG, Tet32, Tet40, TetO, TetQ and TetW, were found in all 162 samples from the three populations ( Supplementary Table S3 and Supplementary Fig. S3 ). The prevalent erythromycin resistance gene type ErmB, previously identified in faecal metagenomic DNA [9] , was found in 161 of 162 samples. Overall, 70 resistance gene types appeared in more than 50% of individuals in the Chinese population, while 45 and 49 types in more than 50% of Danish and Spanish individuals, respectively ( Supplementary Fig. S3 ). Interestingly, TcR genes encoding Tet37, a novel gene type originally identified from oral metagenome [18] , was present in nearly 94% individuals, indicating that this resistance gene type is prevalent in the human gut. Moreover, genes encoding a new type of ribosome protection protein associated with TcR, Tet36, which was first identified in a tetracycline-resistant Bacteroides strain from swine manure pits in the United States [19] , were found in nearly 16% of Chinese individuals. However, these genes were not found in Danish or Spanish individuals, and it will be interesting to investigate why genes of this type are so prevalent in the guts of Chinese people. Abundance of the resistance genes in China is the highest To compare the abundances of antibiotic resistance genes in the Chinese, Danish and Spanish populations, we computed the relative enrichment of each of the genes based on sequencing coverage by using the original Illumina GA short reads (see Methods). On average, the resistance genes accounted for 0.94, 0.44 and 0.89% of the total gut genes in Chinese, Danish and Spanish individuals, respectively ( Fig. 1 ); three Spanish inflammatory bowel disease (IBD) samples, V1.UC-14, O2.UC-16 and O2.UC-18, showed much higher ratio of resistance genes in the gut, ranging from 1.89 to 2.73%. When these three outliers were removed, the average abundance of antibiotic resistance genes in the Spanish population was reduced to 0.76%. Both the Chinese and Spanish individuals presented a significant higher number of resistance genes than the Danish individuals (Mann–Whitney test, P =5.4E−15 and 1.6E−11, respectively). 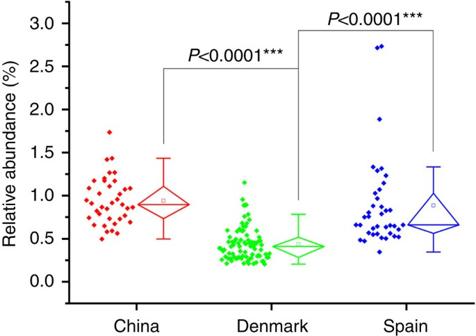Figure 1: Comparison of the relative abundance of the total antibiotic resistance genes in each individual. See the Methods section for the detailed calculation process. The diamond boxes on the right denote the interquartile range (IQR) between the first and third quartiles (25th and 75th percentiles, respectively), and the line and the square inside the boxes denote the median and mean, respectively. The whiskers denote the lowest and highest values within 1.5 times the IQR from the first and third quartiles, respectively. The samples are shown as dots on the left. The asterisks on the top indicateP<0.0001 (Mann–Whitney test). China:n=38; Denmark:n=85; Spain:n=39. Outliers in this figure were not used for comparative analysis inFig. 5andSupplementary Fig. S5. Figure 1: Comparison of the relative abundance of the total antibiotic resistance genes in each individual. See the Methods section for the detailed calculation process. The diamond boxes on the right denote the interquartile range (IQR) between the first and third quartiles (25th and 75th percentiles, respectively), and the line and the square inside the boxes denote the median and mean, respectively. The whiskers denote the lowest and highest values within 1.5 times the IQR from the first and third quartiles, respectively. The samples are shown as dots on the left. The asterisks on the top indicate P <0.0001 (Mann–Whitney test). China: n =38; Denmark: n =85; Spain: n =39. Outliers in this figure were not used for comparative analysis in Fig. 5 and Supplementary Fig. S5 . Full size image We then compared antibiotic resistance gene abundance between Spanish healthy individuals and the IBD patients. Except the three samples exhibiting extremely high ratios of resistance genes, which was probably caused by the recent usage of antibiotics, the remaining 22 IBD samples did not display statistical difference with healthy individuals in antibiotic resistance gene abundance (Mann–Whitney test, P =0.974, Supplementary Fig. S4 ). Therefore, to gain the full profile of antibiotic resistance genes in the Spanish population, the IBD samples were still used in the following analysis. Resistance gene abundance and SNPs are regionally different A hierarchical clustering tree was constructed based on the relative abundance of each resistance gene type, while 150 other functional categories (clusters of orthologous groups (COGs)) were randomly selected (nine times sampling) for clustering (used as control). The results indicated that most individuals from the three countries could be clustered in separated groups by using antibiotic resistance genes but less represented by using other functional genes ( Fig. 2 , Supplementary Figs S5 and S6 ). It implied that the distribution of antibiotic resistance genes and their abundance are geographically different. A total of 21 gene types with a relative abundance of more than 10 −5 were present in at least 60% of individuals, and more than one-third of these gene types were TcR genes. 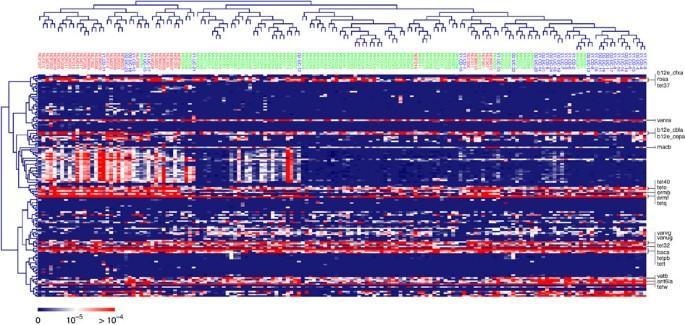Figure 2: Heat map of the relative abundance of each gene type in each individual and hierarchical clustering. The sample identifiers for Chinese, Danish and Spanish individuals are coloured in red, green and blue, respectively. The gene types (rows) and samples (columns) were clustered with the MultiExperiment Viewer (MeV version 4.6) using the Spearman rank correlation and complete linkage. Gene types with a relative abundance of >10−5present in at least 60% of individuals are listed on the right. The indicator on the bottom denotes the relationship between the relative abundance and colour range. Figure 2: Heat map of the relative abundance of each gene type in each individual and hierarchical clustering. The sample identifiers for Chinese, Danish and Spanish individuals are coloured in red, green and blue, respectively. The gene types (rows) and samples (columns) were clustered with the MultiExperiment Viewer (MeV version 4.6) using the Spearman rank correlation and complete linkage. Gene types with a relative abundance of >10 −5 present in at least 60% of individuals are listed on the right. The indicator on the bottom denotes the relationship between the relative abundance and colour range. Full size image The SNPs on antibiotic resistance genes detected in the Chinese population were different from those in the European population, as reflected in the neighbour-joining tree ( Fig. 3 ). The Danish and Spanish populations could not be clustered separately based on these SNPs. The reasons for this may be complex and diverse. We assume that the antibiotic resistance gene variants could be partly attributed to the altered microbiota by differences of population structure or different antibiotic usage in the two continents where the three countries reside. 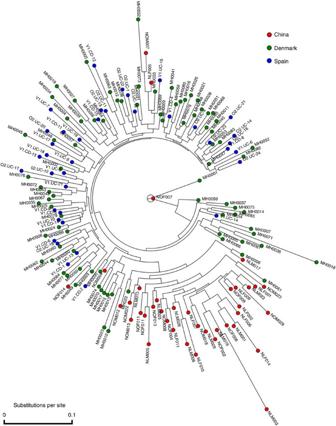Figure 3: The neighbour-joining tree obtained using the SNPs in antibiotic resistance genes from the 162 samples. The tree was constructed using PHYLIP (Methods). Red, green and blue dots denote Chinese, Danish and Spanish individuals, respectively. Figure 3: The neighbour-joining tree obtained using the SNPs in antibiotic resistance genes from the 162 samples. The tree was constructed using PHYLIP (Methods). Red, green and blue dots denote Chinese, Danish and Spanish individuals, respectively. Full size image Representative resistance gene types in different countries The top ten most abundant gene types varied from country to country; however, TetQ was the most abundant type in all three countries ( Fig. 4 and Supplementary Fig. S7A ). Previous work also indicated that, over the past 3 decades, the prevalence of the TetQ gene has increased from being carried in ~30 to more than 80% of Bacteriodes isolates, most likely due to horizontal gene transfer [20] . Another study showed that TetW genes were the most prevalent TcR genes in faecal metagenomic DNA, as identified through microarray analysis [9] . Here, we revealed that TetW gene abundance differs from country to country and were ~13 and 3 times less abundant than TetQ genes in the Chinese and Spanish populations, respectively, whereas the abundances of these two gene types were nearly the same in the Danish population. 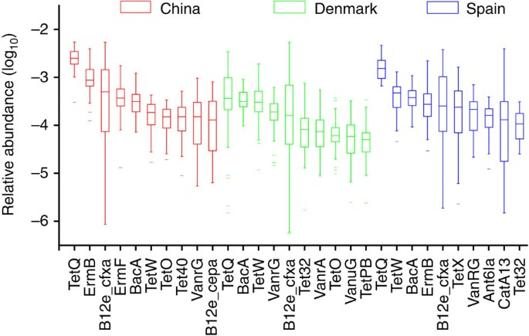Figure 4: Comparison of the top ten most abundant antibiotic resistance gene types in the different populations. Boxes denote the interquartile range (IQR) between the first and third quartiles (25th and 75th percentiles, respectively), and the line inside the boxes denotes the median. The whiskers denote the lowest and highest values within 1.5 times the IQR from the first and third quartiles, respectively. Figure 4: Comparison of the top ten most abundant antibiotic resistance gene types in the different populations. Boxes denote the interquartile range (IQR) between the first and third quartiles (25th and 75th percentiles, respectively), and the line inside the boxes denotes the median. The whiskers denote the lowest and highest values within 1.5 times the IQR from the first and third quartiles, respectively. Full size image The MLS (macrolides, lincosamides and streptogramin) resistance gene type ErmB was the second and the fourth most abundant gene type in the Chinese and Spanish populations, respectively, but was not among the top ten most abundant gene types from Denmark population ( Fig. 4 ). However, among all Erm types, ErmB was the most common gene type in any country, followed by ErmF and ErmG (the three major types) ( Supplementary Fig. S7B ). A beta-lactamase gene type, Bl2e_cfxa, conferring resistance to cephalosporin, was also very common in every population, but its abundance differed greatly from individual to individual ( Fig. 4 ); Bl2e_cfxa, Bl2e_cepa and Bl2e_cbla are the three major antibiotic resistance gene types for cephalosporins ( Supplementary Fig. S7C ). The bacitracin resistance gene type, BacA, was found at a very high relative abundance in each population; the abundance of this gene type was nearly the same among the different populations ( Fig. 4 ). This gene has recently been renamed UppP, corresponding to an undecaprenyl pyrophosphate phosphatase [21] , which may be intrinsic in bacteria, as its homologues can be found in 153 genera (ARDB). VanRG (together with VanSG and VanYG) encodes a putative regulatory system (a component of the vancomycin-resistant VanG-type operon) and was also very abundant. As not all structural gene sequences of individual Van-type operons (at least five genes for each Van operon) can be assembled together, it is difficult to estimate the true abundance of the individual Van operons. However, most of the structural genes of all six known vancomycin resistance operons were found in each population ( Supplementary Fig. S8 ). Among all Van types, the VanG operon structural genes are the most common in each sample, and a total of 87 individuals exhibited all eight structural genes of the VanG operon, indicating the existence of a potential complete VanG operon in these samples. In addition, we found a complete sequence for the VanB operon, including seven structural genes, on the scaffold of a Danish sample, MH0012. TcR genes are the most abundant in human gut microbiota We mapped each antibiotic resistance gene type to its corresponding antibiotic according to WHO ATC code J01, and the relative abundances of types conferring resistance to the same antibiotic were summed ( Fig. 5 ). The results showed that antibiotic resistance genes of three antibiotic classes, tetracyclines, MLSs and beta_lactams, accounted for >75% of the total antibiotic resistance genes in each of the three countries, and the TcR genes were the most abundant, which accounted for nearly 50% of all resistance genes ( Fig. 5 ). The high abundance of TcR genes was further confirmed through functional screening of resistant clones from the fosmid libraries of three healthy Chinese individuals. Among 100 drug-resistant fosmid clones, 74 clones were resistant to tetracycline, 14 to gentamicin and 12 to amoxicillin ( Supplementary Table S4 ). 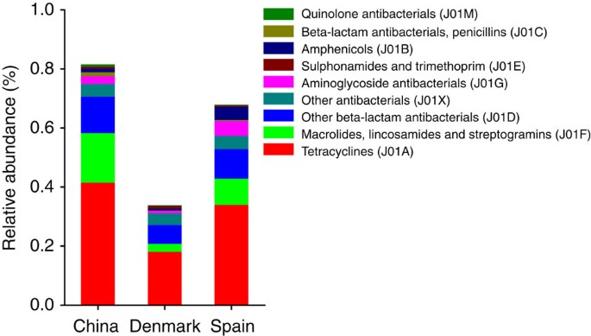Figure 5: The relative abundance of antibiotic resistance gene types assigned to each major antibiotic class in the different populations. Resistance gene types were mapped to antibiotics according to the ARDB, and the classification of antibiotics was based on WHO ATC code J01. The average abundance for each gene type among individuals was used for mapping (excluding outliers). Resistances determined by more than one gene are not included, for example, by the vancomycin resistance operon. China:n=37; Denmark:n=80; Spain:n=36. Figure 5: The relative abundance of antibiotic resistance gene types assigned to each major antibiotic class in the different populations. Resistance gene types were mapped to antibiotics according to the ARDB, and the classification of antibiotics was based on WHO ATC code J01. The average abundance for each gene type among individuals was used for mapping (excluding outliers). Resistances determined by more than one gene are not included, for example, by the vancomycin resistance operon. China: n =37; Denmark: n =80; Spain: n =36. Full size image Our results provide a comprehensive overview of the antibiotic resistance gene reservoir in the human gut microbiota at the metagenomic level. It is recognized that antibiotic consumption is the main cause of the emerging resistance, and differences in drug resistance in the three countries may have been attributed to the differential selection pressures of antibiotics [22] . In China, the overuse of antibiotics and antibiotic resistance are severe. Approximately 75% of patients with seasonal influenza are estimated to be prescribed antibiotics [23] . In addition, China exhibits the most rapid growth rate of drug resistance compared with Kuwait and the United States [24] . These factors may partly explain why Chinese people harbour the highest number of resistance genes in their gut, though we do not know exactly how these resistance genes were acquired and transmitted. On the other hand, it should be noted that the relation between antibiotic resistance genes and the usage of antibiotics is very complex. The contribution to the enrichment of antibiotic resistance genes may not be only by the antibiotic abuse. There are some intrinsic mechanisms that can give rise to drug resistance. For example, efflux pumps were originally reported as being involved in signal trafficking or resistance to toxic compounds, but it can involve in the efflux of antibiotics as well [25] . Moreover, antibiotic resistance can be selected by heavy metals [26] , and this phenomenon has been observed in the human gastrointestinal tract [27] . Furthermore, antibiotic use in animals may contribute to the emerging of antibiotic resistance in humans, that is, antibiotic-resistant bacteria and antibiotic resistance genes can spread from animals to humans through many routes such as food chain [28] , [29] . Recent work also found that exchange of antibiotic resistance genes between bacteria from farm animals, human food and human-associated bacteria (clinical isolates, and so on) by horizontal gene transfer, which can explain some antibiotic resistance genes, may come from animal source [30] . At last, antibiotic resistance genes are known to have seasonal oscillations especially in natural environments, river, for example [31] . However, to what extent the human gut antibiotic resistance genes were affected by such factors should be further addressed. Nevertheless, it is noteworthy that the batch effect of sampling could be factors that may influence the outcome of studies on human gut microbiomes [32] . Although gut samples from three different populations used in this study were obtained by following the similar protocols and using the same sequencing platforms, batch effects may still exist owing to multi-site sampling. In addition, the amount of samples is relatively limited to reflect the antibiotic resistance gene profile of the entire populations owing to the sequencing capability and affordability. Therefore, large-scale study is needed to have a better understanding of antibiotic resistance genes in human gut microbiota. These would help to determine whether antibiotic resistance genes carried by human gut commensals pose a risk, for example, of horizontal transfer to potentially pathogenic microbes. Note added in proof: During the preparation of this manuscript, Forslund et al. published results using metagenomic datasets of human gut microbiota from individuals residing in Spain, Denmark and the United States. They demonstrate that antibiotics used in animal husbandry and the long-term use of antibiotics are the strongest determinants of the antibiotic resistance genes repertoire in the human gut microbiome [33] . Data sets The metagenomic data set from 124 European and 38 Chinese samples was generated in previous studies [17] , [34] ; original data are available to download from BGI website ( http://gutmeta.genomics.org.cn/ ) and NCBI SRA database (accession number: SRA045646), respectively. In the type 2 diabetes gut microbiota study [34] , a total of 345 Chinese individuals’ gut samples were sequenced in two stages. The 38 Chinese samples we used here were a part of healthy samples completed in the first stage. The construction of the human gut non-redundant gene set was performed as previously described [17] . Publicly available metagenomic data sets from Sargasso Sea Bacterioplankton Community (MG-RAST Project ID: mgp47), Waseca County Farm Soil Metagenome (mgp8), Mediterranean Bathypelagic Metagenome (mgp3), Alvinella Pompejana Epibiont Metagenome (mgp4), Antarctica Aquatic Microbial Metagenome (mgp20), Rain Forest Soil Microbial Communities (mgp45), Lake Erie Bloom Metagenome (mgp715) and Ocean Drilling Program (mgp470) were downloaded from MG-RAST server [35] ( http://metagenomics.anl.gov/ ). All of the antibiotic resistance genes were from the (version 1.1) ( http://ardb.cbcb.umd.edu/ ). Annotated protein sequences in UniProtKB/SwissProt were downloaded from UniProt ( http://www.uniprot.org/ ). BLAST searches for antibiotic resistance genes A command-line version of resistance genes annotation tool together with a core set of 7825 antibiotic resistance proteins was downloaded from the ARDB. All non-redundant genes in each metagenomic data set were aligned with these resistance proteins using BLASTx with an E -value threshold of 1e−10 and query coverage of at least 70%. To determine the threshold for antibiotic resistance gene BLAST search, the manually curated UniProtKB/SwissProt database was used as test data. We aligned all sequences in SwissProt with ARDB and summarized the receiver operating characteristic and precision/recall rate at different similarity cutoff levels (90, 80, 70 and 60%) according to the consistency of annotations between SwissProt and ARDB ( Supplementary Data 1 and Supplementary Fig. S1 ). Taxonomic affiliation The taxonomic affiliation analysis of antibiotic resistance genes in the human gut was based on the use of the MEtaGenome Analyzer (MEGAN, version 3.9) [36] . Before applying this programme, sequences were compared against NCBI nr databases using BLASTx under the default parameters. MEGAN was then used to compute and interactively explore the taxonomic content of the data set, employing the NCBI taxonomy feature to summarize and order the results (LCA parameters: mini-score 35, top percentage 10%). Determination of relative gene abundance The gene abundance was determined by using the method similar to RPKM (reads per kilo bases per million reads) used for quantifying gene expression from RNA sequencing data. In brief, high-quality original Illumina GA read pairs from each human gut sample were aligned with the non-redundant gene set using SOAP [37] . For each gene, Gi, the number of read pairs that aligned to it divided by the length of the gene was calculated as Num_Gi, and the relative abundance, RNum_Gi, of each gene in each sample ( n genes) was computed using the following formula: RNum_Gi=Num_Gi/∑ i =1 n Num_Gi. The sum of the relative abundance of each antibiotic resistance gene mapped to the same gene type (according to the ardbAnno mapping file in ARDB) was defined as the gene type’s relative abundance ( Supplementary Data 2 ). Hierarchical clustering of samples and gene types was performed based on the relative abundance of the gene types using the MultiExperiment Viewer (MeV version 4.6) with the Spearman rank correlation and complete linkage. To validate the clustering result, genes were randomly selected by their COG assignment and used as control (nine times sampling, each time 150 COGs). We then calculated the tree distance (PHYLIP symmetric difference) between antibiotic resistance gene type clustering and COGs clustering, and distance between each COGs clustering. Mann–Whitney test was used for statistical comparisons between these two groups. SNP-based neighbour-joining tree First, we identified the SNPs present in 1,093 antibiotic resistance genes from 162 samples under the criteria minor allele frequency>0.02, depth≥100. Next, a total of 527 SNPs that were present in at least 50% of the samples were selected for phylogenetic tree construction. Calculation of the distance between two individuals was conducted as follows: (A) T bases : statistic representing the number of loci shared by these two individuals; (B) D bases : statistic representing the number of loci of including the base-type diversity in the two individuals; and (C) Dist= D bases / T bases : the genetic distance between the two individuals. Finally, an NJ tree was built according to the genetic distances between all of the individuals’ using PHYLIP. Functional screening of antibiotic-resistant fosmid clones Faecal samples were obtained from three healthy unrelated volunteers. All of these subjects had not used antibiotics for at least 6 months before sampling. Isolation of DNA from the gut microbiomes was performed as described previuously [38] by using a 1 g faecal sample instead of a soil sample. DNA purification was conducted via pulsed-field gel electrophoresis and gel electrophoresis using the CHEF-DRIII system (Bio-Rad), as described by Hu [39] . Fosmid libraries were constructed using the CopyControl HTP fosmid library production kit (Epicentre) according to the manufacturer’s instructions. The repaired DNA was ligated into the pCC2FOS fosmid vector (Epicentre), and the ligated DNA mixtures were packaged using the supplied lambda packaging extracts and transformed into an EPI300-T1 R phage T1-resistant E. coli host. All three libraries (total size of 200,000 clones) were amplified by plating onto LB agar plates containing chloramphenicol (12.5 μg ml −1 ), and colonies were then recovered from the plates and mixed together. For functional selection, a onefold coverage of the library, corresponding to 200,000 clones, was plated on LB agar plates containing binary combinations of chloramphenicol (12.5 μg ml −1 ) and one representative antibiotic from each of the three major classes (tetracyclines, aminoglycosides and beta_lactams) ( Supplementary Table S4 ), then incubated at 37 °C for 24 h. How to cite this article: Hu, Y. et al. Metagenome-wide analysis of antibiotic resistance genes in a large cohort of human gut microbiota. Nat. Commun. 4:2151 doi: 10.1038/ncomms3151 (2013).